Engineering the type III secretion system in non-replicating bacterial minicells for antigen delivery Type III protein secretion systems are being considered for vaccine development as virtually any protein antigen can be engineered for delivery by these nanomachines into the class I antigen presentation pathway to stimulate antigen-specific CD8 + T cells. A limitation in the use of this system is that it requires live virulence-attenuated bacteria, which may preclude its use in certain populations such as children and the immunocompromised. Here we report the engineering of the Salmonella Typhimurium type III secretion system in achromosomal, non-replicating nanoparticles derived from bacterial minicells. The engineered system is shown to be functional and capable of delivering heterologous antigens to the class I antigen presentation pathway stimulating immune responses both in vitro and in vivo . This antigen delivery platform offers a novel approach for vaccine development and cellular immunotherapy. Efficient vaccines must not [1] , [2] only stimulate innate immune receptors, but also deliver antigens to specific subcellular compartments so that they can be processed via the class I and class II antigen-presenting pathways resulting in the production of antigen-specific cytotoxic T cells and antibodies [3] . Live-replicating pathogenic bacteria, such as Salmonella Typhimurium, rendered avirulent and engineered with the ability to express foreign antigens are being considered as vaccine vectors to protect against various infectious diseases or as therapeutic agents against cancer [4] , [5] , [6] . Although they potently stimulate innate immune receptors, one limitation of these bacterial vaccine platforms is their inefficient capacity to stimulate cytotoxic T-cell responses [7] , [8] , which require the delivery of antigens to the cytosol of antigen-presenting cells. This limitation has been largely overcome by the use of type III secretion systems (T3SS) [1] , [2] , which are complex multi-protein molecular machines that deliver bacterial virulence effector proteins into the host cell cytosol [9] . Proteins destined to travel the T3SS pathway possess discrete signals that direct them to the secretion machine [10] . When incorporated into heterologous proteins, these signals can target virtually any protein for delivery through this secretion pathway [2] , [11] . Consequently, T3SS have been engineered to deliver heterologous antigens in the context of virulence-attenuated bacterial pathogens [1] . Heterologous protein antigens delivered by this system have been shown to stimulate antigen-specific CD8 + T cells, which in animal models conferred protection to a variety of infectious diseases or caused the regression of established tumors [1] , [12] , [13] , [14] , [15] , [16] , [17] , [18] , [19] , [20] , [21] . A second limitation of the virulence-attenuated bacterial vaccine platforms relates to their safety. Residual virulence of the attenuated pathogen or the potential for virulence-reversion may limit their use in certain populations such as children or the immunocompromised. To overcome some of the limitations of virulence-attenuated bacterial antigen delivery vectors while retaining some of its benefits, we sought to engineer the T3SS in a non-replicating antigen-delivery platform. As protein translocation by T3SSs requires energy provided by ATP hydrolysis and a proton gradient [22] , the use of this system has been restricted to the context of live virulence-attenuated bacteria. The intrinsic complexity of the assembly of this large, multi-protein machine combined with its energy requirements, virtually preclude the development of a synthetic platform capable of supporting the function of T3SS. As an alternative to a synthetic platform, we sought to engineer bacterial minicells with the capacity to deliver heterologous proteins through the S. Typhimurium T3SS encoded within its pathogenicity island 1 (SPI-1). Bacterial minicells result from aberrant cell division and although they lack chromosomal DNA they have the capacity to synthesize proteins and sustain a proton gradient [23] . In addition, these nanoparticles have immune adjuvant capacity [24] as they retain most of the bacterial components capable of stimulating innate immune receptors [25] . We report here the assembly of a functional T3SS in bacterial minicells and its use for antigen delivery. Bacterial minicells assemble T3SS We isolated minicells from a S. Typhimurium strain carrying a deletion mutation in minD ( Supplementary Fig. S1 ), which is required for proper cell division [26] . Loss of this gene results in aberrant cell division with the production of a large number of minicells ( Fig. 1a ). We examined by LC-MS/MS highly purified minicell preparations for the presence of components of the SPI-1 T3SS. Although we were able to detect most of the SPI-1 T3SS components ( Fig. 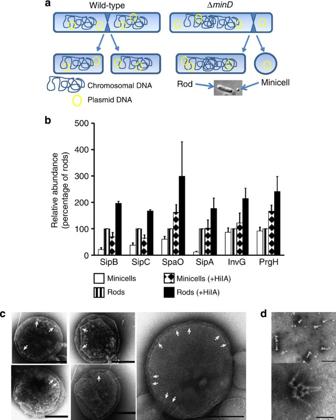Figure 1: Bacterial minicells assemble a type III secretion system. (a) Schematic of minicell generation (see alsoSupplementary Fig. S1). (b) Relative abundance of selected T3SS proteins analysed by immunoblotting. Values are standardized compared with those obtained from wild-typeS.Typhimurium rods and normalized according to the total protein concentration of each sample. Values are the mean±s.d. of three independent measurements. See additional information in Methods andSupplementary Figs S2,S3. (c) Electron micrographs of negatively stained osmotically shocked minicells. Arrows indicate T3SS needle complexes on the minicell envelope. Scale bars, 200 nm. (d) Electron micrographs of negatively stained needle complexes isolated from purified minicells. Scale bars, 100 nm (top) and 50 nm (bottom). 1b , Table 1 , and Supplementary Table S1 ), the concentrations of T3SS-associated proteins were significantly lower compared with that of the originating bacterial cells. In particular, the protein translocases, which mediate the passage of the type III secreted proteins through the mammalian cell membrane [27] , were significantly depleted in bacterial minicells. These results were confirmed by western blot analysis of selected T3SS-associated proteins ( Fig. 1b ; Supplementary Figs S2,S3a ). These findings indicated that although components of the SPI-1 T3SS can partition into minicells, they might not be abundant enough to efficiently function as a protein delivery machine. To increase the levels of SPI-1 T3SS components partitioned into minicells, we introduced into the S. Typhimurium minD strain a plasmid encoding HilA, the positive transcription regulator of the SPI-1 T3SS, expressed under a rhamnose-inducible promoter [28] . Previous studies have shown that the overexpression of HilA results in increased levels of all components of this system. LC-MS/MS analysis of minicells produced by this strain showed significantly increased levels of SPI-1 T3SS components ( Fig. 1b , Table 1 ; Supplementary Fig. S2,S3a and Supplementary Table S2 ). Consistent with these findings, minicells assembled T3SS needle complexes, the core structure of this secretion machine [29] , which could be readily visualized by electron microscopy in intact minicells ( Fig. 1c ) or in purified needle complex preparations ( Fig. 1d ). These results indicate that SPI-1 T3SS components not only can partition into minicells but also can assemble into a potentially functional secretion machine. Figure 1: Bacterial minicells assemble a type III secretion system. ( a ) Schematic of minicell generation (see also Supplementary Fig. S1 ). ( b ) Relative abundance of selected T3SS proteins analysed by immunoblotting. Values are standardized compared with those obtained from wild-type S. Typhimurium rods and normalized according to the total protein concentration of each sample. Values are the mean±s.d. of three independent measurements. See additional information in Methods and Supplementary Figs S2,S3 . ( c ) Electron micrographs of negatively stained osmotically shocked minicells. Arrows indicate T3SS needle complexes on the minicell envelope. Scale bars, 200 nm. ( d ) Electron micrographs of negatively stained needle complexes isolated from purified minicells. Scale bars, 100 nm (top) and 50 nm (bottom). Full size image Table 1 Relative levels of T3SS-associated proteins in purified minicells. Full size table Minicells assemble functional T3SS A functional SPI-1 T3SS machine must be able to deploy the protein translocases SipB, SipC and SipD, which will eventually mediate the passage of the secreted proteins through the mammalian cell membrane [27] . Before contact with host cells, only SipD, a component of the needle tip complex, is displayed on the bacterial surface [30] . To probe for the presence of potentially functional T3SS complexes, we examined minicells by immunofluorescence microscopy for the presence of surface-localized SipD. We found that a significant proportion of minicells isolated from bacterial cells overexpressing HilA displayed SipD on their surface ( Fig. 2a ). In contrast, minicells isolated from a SPI-1 T3SS-defective mutant did not ( Fig. 2a ). These results indicate that minicells assemble T3SS complexes potentially competent for protein translocation into mammalian cells. 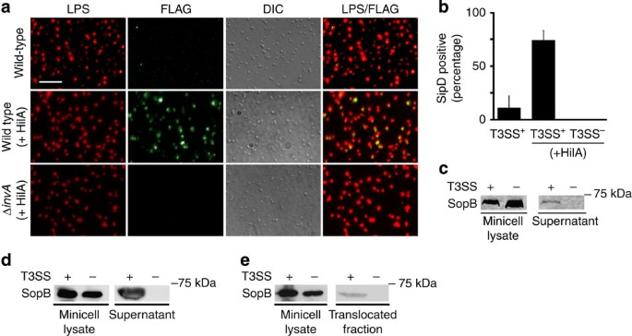Figure 2: The type III secretion system in minicells is functional. (a,b) Detection of the needle complex tip protein SipD on the surface of purified minicells. Minicells were isolated from wild-type or T3SS-defective (ΔinvA)S.Typhimurium strains expressing SipD-FLAG and carrying a plasmid expressing the SPI-1 T3SS-positive transcriptional regulator HilA. Minicells were stained with an antibody to LPS (red), an antibody against the FLAG tag (green), and examined by immunofluorescence and DIC microscopy. Scale bar, 2.5 μm (a). The % of minicells showing surface SipD stain is shown in (b). Values represent the mean±s.d. of three independent experiments in which a minimum of 4,000 cells per strain were counted. (c,d) Secretion ofde novosynthesized effector proteins by purified minicells through their SPI-1 T3SS. Minicells were isolated from wild-type or T3SS-defective (ΔinvA)S.Typhimurium strains carrying a plasmid encoding the SPI-1 T3SS effector SopB expressed under the control of an arabinose-inducible promoter. Isolated minicells were incubated for 3 h in the presence of arabinose and the presence of SopB in minicell lysates and supernatants were analysed by western blot (c). Alternatively, minicells were exposed to cultured Henle-407 cells and the presence of SopB in supernatants examined as described above (d). (e) Minicell-mediated, type III secretion-dependent protein translocation into cultured epithelial cells. Henle-407 cells were treated with minicells isolated from type III secretion competent or type III secretion-defective (ΔinvA) as described above and added to Henle-407 cells for 2.5 h. The presence of the effector protein SopB in minicell lysates and the translocated fraction was assayed by western blot. Figure 2: The type III secretion system in minicells is functional. ( a , b ) Detection of the needle complex tip protein SipD on the surface of purified minicells. Minicells were isolated from wild-type or T3SS-defective (Δ invA ) S. Typhimurium strains expressing SipD-FLAG and carrying a plasmid expressing the SPI-1 T3SS-positive transcriptional regulator HilA. Minicells were stained with an antibody to LPS (red), an antibody against the FLAG tag (green), and examined by immunofluorescence and DIC microscopy. Scale bar, 2.5 μm ( a ). The % of minicells showing surface SipD stain is shown in ( b ). Values represent the mean±s.d. of three independent experiments in which a minimum of 4,000 cells per strain were counted. ( c , d ) Secretion of de novo synthesized effector proteins by purified minicells through their SPI-1 T3SS. Minicells were isolated from wild-type or T3SS-defective (Δ invA ) S. Typhimurium strains carrying a plasmid encoding the SPI-1 T3SS effector SopB expressed under the control of an arabinose-inducible promoter. Isolated minicells were incubated for 3 h in the presence of arabinose and the presence of SopB in minicell lysates and supernatants were analysed by western blot ( c ). Alternatively, minicells were exposed to cultured Henle-407 cells and the presence of SopB in supernatants examined as described above ( d ). ( e ) Minicell-mediated, type III secretion-dependent protein translocation into cultured epithelial cells. Henle-407 cells were treated with minicells isolated from type III secretion competent or type III secretion-defective ( ΔinvA ) as described above and added to Henle-407 cells for 2.5 h. The presence of the effector protein SopB in minicell lysates and the translocated fraction was assayed by western blot. Full size image Minicells are metabolically active and capable of synthesizing de novo plasmid-encoded proteins after the partitioning of plasmids into minicells [23] . We therefore tested whether purified minicells were competent for the secretion and translocation into cultured mammalian cells of a de novo synthesized SPI-1 T3SS effector protein. Minicells were isolated from T3SS-competent or T3SS-defective strains carrying a plasmid, which encodes the effector protein SopB [31] expressed from an arabinose-inducible promoter. Isolated minicells were incubated in the presence of arabinose for 3 h and the secretion of SopB to culture medium was assessed by western immunoblot analysis. SopB was detectable in supernatants of T3SS-competent minicells but not from supernatants of T3SS-defective minicells despite equivalent amount of SopB in lysates of whole minicells obtained from either strain ( Fig. 2c and Supplementary Fig. S3b ). One of the characteristic features of some T3SSs such as the one encoded by the S. Typhimurium SPI-1 is that their activity is stimulated upon contact with eukaryotic cells [32] . Consistent with this behaviour, we found greater levels of secreted SopB upon exposure of minicells to cultured Henle-407 epithelial cells ( Fig. 2d ). We also examined the ability of minicells to inject proteins into cultured epithelial cells using a fractionation protocol previously developed in our laboratory to detect translocated effector proteins in the cytosol of infected cells [27] . We found detectable levels of translocated SopB in preparation of cultured cells exposed to minicells obtained from wild-type S. Typhimurium but not in those exposed to minicells obtained from a SPI-1 T3SS-defective mutant ( Fig. 2e ). These results indicate that minicells assemble a functional T3SS capable of mediating protein secretion and translocation into eukaryotic cells. T3SS in minicells can deliver antigen in vitro It has been previously shown that live, virulence-attenuated S. Typhimurium can deliver heterologous antigens in a T3SS-dependent manner to the major class I antigen presentation pathway [1] . To determine whether the T3SS in minicells was also capable of such delivery, the first 104 amino acids of SopE, containing the T3SS-targeting signal [19] , were fused to 16 amino acids of the OVA antigen containing the class I-restricted SIINFEKL peptide [33] along with a C-terminal 3xFLAG tag (SopE-OVA) ( Fig. 3a ). A plasmid encoding this chimeric protein was introduced into minicell-producing T3SS-competent or T3SS-defective S. Typhimurium strains ( Fig. 3b and Supplementary Fig. S3c ). We then tested the ability of minicells to deliver SopE-OVA in a T3SS-dependent manner to the class I antigen-presenting pathway. Murine RMA cells were incubated with minicells purified from different parental strains and the ability of the RMA cells to present the class I-restricted OVA peptide to the class I-restricted B3Z T-cell reporter [34] was assayed by measuring β-galactosidase production by the reporter cells. Minicells purified from T3SS-competent S. Typhimurium were found to efficiently deliver SopE-OVA to RMA cells ( Fig. 3c ). In contrast, minicells obtained from a T3SS-defective mutant were not ( Fig. 3c ). These results demonstrate that minicells are capable of T3SS-dependent translocation of an effector-antigen construct. In addition, these results indicate that minicell T3SS-delivered effector-antigen constructs can elicit a MHC class I-restricted immune response and activation of CD8 + T-cells in vitro . 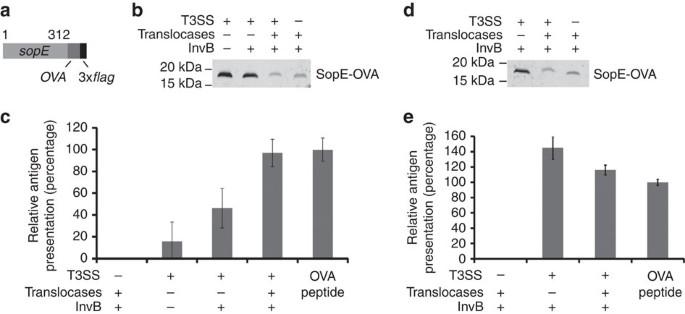Figure 3: T3SS-dependent antigen delivery by minicellsin vitro. (a) Schematic of the SopE-OVA construct used in these studies. (b) Western blot analysis of minicells obtained from wild-type or T3SS-defective (ΔinvA)S.Typhimurium strains expressing the SopE-OVA construct and used in the experiment shown in (c). When indicated, the SopE-OVA construct was co-expressed with the SopE chaperone InvB and the T3SS protein translocases and their chaperones to improve protein secretion and/or translocation. Equal amount of total protein was loaded in each sample. (c) Analysis of antigen delivery by minicells to antigen-presenting cells. RMA cells (C57BL/6 mouse hybridomas) were pulsed for 3 h with minicells isolated from wild-type or T3SS-defective (ΔinvA)S.Typhimurium strains. After pulsing, RMA cells were fixed, and used as APCs in a B3Z T-cell activation assay as described in experimental procedures. Values represent the levels of antigen presentation based on the β-galactosidase activity detected in the B3Z T-cell hybridoma reporter and are normalized relative to the values of the OVA peptide-positive control, which was considered 100%. The values are the mean±s.d. of three independent experiments. (d,e) Minicells can deliver antigen to DCsex vivo. (d) Western blot analysis of minicells obtained from wild-type or T3SS-defective (ΔinvA)S.Typhimurium strains expressing the SopE-OVA construct and used in the experiment shown in (e). Equal amount of total protein was loaded in each sample. (e) Bone marrow-derived DCs were pulsed for 3 h with minicells isolated from the indicatedS.Typhimurium strains carrying a plasmid expressing SopE-OVA and the indicated SPI-1 T3SS-associated proteins. After pulsing, DCs were fixed and used as APCs in a B3Z T-cell activation assay as described inSupplementary Materials. Values represent the levels of antigen presentation based on the β-galactosidase activity detected in the B3Z T-cell hybridoma reporter and they are normalized relative to the values of the OVA peptide-positive control, which was considered 100%. The values are the mean±s.d. of two independent experiments. Figure 3: T3SS-dependent antigen delivery by minicells in vitro . ( a ) Schematic of the SopE-OVA construct used in these studies. ( b ) Western blot analysis of minicells obtained from wild-type or T3SS-defective (Δ invA ) S. Typhimurium strains expressing the SopE-OVA construct and used in the experiment shown in ( c ). When indicated, the SopE-OVA construct was co-expressed with the SopE chaperone InvB and the T3SS protein translocases and their chaperones to improve protein secretion and/or translocation. Equal amount of total protein was loaded in each sample. ( c ) Analysis of antigen delivery by minicells to antigen-presenting cells. RMA cells (C57BL/6 mouse hybridomas) were pulsed for 3 h with minicells isolated from wild-type or T3SS-defective (Δ invA ) S. Typhimurium strains. After pulsing, RMA cells were fixed, and used as APCs in a B3Z T-cell activation assay as described in experimental procedures. Values represent the levels of antigen presentation based on the β-galactosidase activity detected in the B3Z T-cell hybridoma reporter and are normalized relative to the values of the OVA peptide-positive control, which was considered 100%. The values are the mean±s.d. of three independent experiments. ( d , e ) Minicells can deliver antigen to DCs ex vivo . ( d ) Western blot analysis of minicells obtained from wild-type or T3SS-defective (Δ invA ) S. Typhimurium strains expressing the SopE-OVA construct and used in the experiment shown in ( e ). Equal amount of total protein was loaded in each sample. ( e ) Bone marrow-derived DCs were pulsed for 3 h with minicells isolated from the indicated S. Typhimurium strains carrying a plasmid expressing SopE-OVA and the indicated SPI-1 T3SS-associated proteins. After pulsing, DCs were fixed and used as APCs in a B3Z T-cell activation assay as described in Supplementary Materials . Values represent the levels of antigen presentation based on the β-galactosidase activity detected in the B3Z T-cell hybridoma reporter and they are normalized relative to the values of the OVA peptide-positive control, which was considered 100%. The values are the mean±s.d. of two independent experiments. Full size image Although purified minicells were shown to be capable of delivering antigen in a T3SS-dependent manner, the efficiency of delivery was relatively poor. We reasoned that this inefficiency might be at least partially due to the lower levels of some critical components of the T3SS in minicells. Secretion of proteins through the T3SS requires customized cytoplasmic chaperones, which target them to the secretion machinery [9] . As proteomic analysis indicated that the partitioning of the SopE chaperone InvB (as well as other T3SS chaperones) into minicells was inefficient ( Supplementary Table S1 ), we added invB to the plasmid expressing the chimeric sopE-OVA construct that partitions into minicells. Expression of invB in tandem with sopE-OVA improved the relative antigen presentation of minicells by over two-fold ( Fig. 3c ). The proteomics analysis also showed that the translocases SipB, SipC and SipD and their associated chaperones InvE and SicA were also depleted in minicells ( Supplementary Table S1 ). Consequently, we added to the expression plasmid the genes encoding these proteins. Although expression of the antigen construct was slightly lower ( Fig. 3b and Supplementary Fig. S3c ), minicells obtained from this strain showed a significantly higher antigen-presenting ability, achieving a level essentially equivalent to that of the peptide-positive control ( Fig. 3c ). These results show that the T3SS-mediated antigen delivery by purified minicells can be optimized by the expression of T3SS components encoded by plasmids that can partition into minicells. Dendritic cell (DC) immunotherapy is emerging as a promising strategy for autologous treatment of infectious diseases and cancer [35] . Some configurations of this strategy involve the ex vivo antigen loading of autologous DCs before their application back to the recipients. Minicells could potentially offer advantages for ex vivo loading of DCs as not only they can deliver antigen to the class I antigen-presenting pathway, essential in anti-tumor immune responses, but also they can potentially deliver DC maturation signals through the Toll-receptor agonists present in these nanoparticles. We therefore tested whether minicells could deliver antigen to DCs ex vivo . Mouse bone marrow-derived DCs were incubated with minicells obtained from strains carrying a plasmid expressing sopE-OVA along with its chaperone invB and the protein translocases and their chaperones ( Fig. 3d and Supplementary Fig. S3d ). Antigen loading was assayed by measuring the ability of DCs to present the class I-restricted OVA peptide to the class I-restricted allogeneic B3Z T-cell reporter cell. We found that the response elicited by the minicell-pulsed DCs in the reporter cell line was equivalent to the peptide-positive control ( Fig. 3e ). Antigen presentation was strictly dependent on the presence of the T3SS in the minicells as DCs pulsed with equivalent number of minicells obtained from a T3SS-deficient bacterial strain did not elicit a response in the reporter cell line ( Fig. 3d and Supplementary Fig. 3d ). These results show that minicells can effectively deliver antigen to DCs ex vivo . T3SS in minicells can prime CD8 + T-cell responses in vivo We evaluated the potential of minicells expressing SopE-OVA to prime CD8 + T-cell responses in vivo . OT-I CD8 + T cells (CD45.2), which can specifically recognize an OVA epitope [36] , were adoptively transferred into C57BL/6J congenic mice expressing CD45.1. Recipient mice were then immunized with purified minicells optimized for the delivery of SopE-OVA by co-expressing the chaperone InvB and the translocases. As controls, mice were immunized with minicells obtained from a T3SS-defective strain expressing SopE-OVA or minicells obtained from a T3SS-competent strain that did not express SopE-OVA ( Fig. 4a and Supplementary Fig. S3e ). After 3 weeks, the recipient mice were boosted with recombinant VSV-OVA and 5 days after the boost mice were killed and the expansion of OT-I CD8 + T-cells was analysed. Mice immunized with minicells purified from the wild-type parental vaccine strain expressing SopE-OVA had a significant expansion of the CD45.2 CD8 + donor OT-I T-cells specific for the OVA peptide ( Fig. 4b ). In contrast, mice immunized with minicells expressing SopE-OVA purified from a T3SS-defective background or minicells lacking SopE-OVA, did not show expansion of the adoptively transferred OT-I CD8 + T-cells upon boosting with VSV-OVA ( Fig. 4b ). These results indicate that minicells can prime antigen-specific CD8 + T-cell responses in vivo in a T3SS-dependent manner. 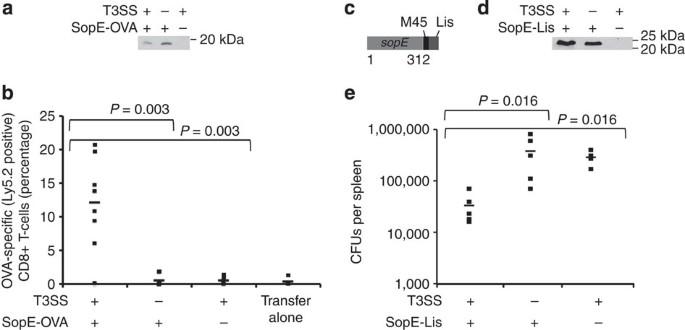Figure 4: T3SS-dependent priming of protective CD8+T-cell responses by minicells. (a) Western blot analysis of minicells obtained from wild-type or T3SS-defective (ΔinvA)S.Typhimurium strains expressing the SopE-OVA construct and used in the experiment shown in (b). Equal amount of total protein was loaded in each sample. (b) Splenocytes from OT-I mice were adoptively transferred into recipient mice (C57BL/6/CD45.1), which were subsequently immunized with minicells isolated from the indicatedS.TyphimuriumΔasdstrains expressing SopE-OVA. Three weeks after minicell immunization mice were boosted and the levels of OVA-specific CD8+T-cells were measured by flow cytometry as indicated in Methods. Values represent the percentage of OVA-specific CD8+T cells in each individual mouse (number of mice used in each category: T3SS+/SopE-OVA+: 9; T3SS−/SopE-OVA+: 7; T3SS+/SopE-OVA−: 7; transfer alone: 4). Data were analysed using the Student’st-test. (c) Schematic of SopE-Lis construct used in the protection experiments. (d) Western blot analysis of minicells obtained from wild-type or T3SS-defective (ΔinvA)S.Typhimurium strains expressing the SopE-Lis construct and used in the experiment shown in (e). (e) BMDCs prepared from Balb/c mice were incubated with minicells isolated from the indicated bacterial strains and transferred by tail vein injection into a Balb/c mouse as indicated in Methods. Six days after transfer mice were challenged withL. monocytogenes, and 3 days after challenge the c.f.u. in spleens were determined (number of mice used in each category: T3SS+/SopE-Lis+: 5; T3SS-/SopE-Lis+: 5; T3SS+/SopE-Lis−: 4). Data were analysed using the Wicoxon rank test. Figure 4: T3SS-dependent priming of protective CD8 + T-cell responses by minicells. ( a ) Western blot analysis of minicells obtained from wild-type or T3SS-defective (Δ invA ) S. Typhimurium strains expressing the SopE-OVA construct and used in the experiment shown in ( b ). Equal amount of total protein was loaded in each sample. ( b ) Splenocytes from OT-I mice were adoptively transferred into recipient mice (C57BL/6/CD45.1), which were subsequently immunized with minicells isolated from the indicated S. Typhimurium Δasd strains expressing SopE-OVA. Three weeks after minicell immunization mice were boosted and the levels of OVA-specific CD8 + T-cells were measured by flow cytometry as indicated in Methods. Values represent the percentage of OVA-specific CD8 + T cells in each individual mouse (number of mice used in each category: T3SS + /SopE-OVA + : 9; T3SS − /SopE-OVA + : 7; T3SS + /SopE-OVA − : 7; transfer alone: 4). Data were analysed using the Student’s t -test. ( c ) Schematic of SopE-Lis construct used in the protection experiments. ( d ) Western blot analysis of minicells obtained from wild-type or T3SS-defective (Δ invA ) S. Typhimurium strains expressing the SopE-Lis construct and used in the experiment shown in ( e ). ( e ) BMDCs prepared from Balb/c mice were incubated with minicells isolated from the indicated bacterial strains and transferred by tail vein injection into a Balb/c mouse as indicated in Methods. Six days after transfer mice were challenged with L. monocytogenes , and 3 days after challenge the c.f.u. in spleens were determined (number of mice used in each category: T3SS + /SopE-Lis + : 5; T3SS - /SopE-Lis + : 5; T3SS + /SopE-Lis − : 4). Data were analysed using the Wicoxon rank test. Full size image We also evaluated the ability of minicells to elicit a protective immune response in a mouse model of Listeria monocytogenes infection. We stimulated ex vivo bone marrow-derived DCs with minicells expressing a chimera consisting of the secretion and translocation domain of SopE fused to Listeria monocytogenes MHC class I-restricted immunogenic peptides from listeriolysin O and p60 (SopE-Lis) ( Fig. 4c ), which have been shown to induce protective CD8 + T-cell responses in Balb/c mice [37] , [38] . For controls, DCs were stimulated ex vivo with purified minicells obtained from a T3SS-defective strain expressing SopE-Lis or minicells obtained from a T3SS-competent strain that did not express SopE-Lis ( Fig. 4d and Supplementary Fig. S3f ). Stimulated DCs were then transferred by tail vein injection into recipient mice, and 6 days after the transfer, recipient mice were challenged with L. monocytogenes . Three days after challenge, mice were killed and the c.f.u. of Listeria mocytogenes in the spleens were enumerated. We found significantly lower number of c.f.u. in the spleens of mice that had received DCs stimulated with T3SS-competent minicells expressing the L. monocytogenes antigens than in the control animals ( Fig. 4e ). These results demonstrate that DCs stimulated ex vivo by T3SS-competent minicells can confer protection from an infectious challenge. We have described here a strategy to engineer the S. Typhimurium T3SS into nanoparticles capable of delivering antigens directly into the cytosol of antigen-presenting cells to stimulate the production of protective, antigen-specific class I-restricted CD8 + T cells. The development of these nanoparticles expands the potential of the T3SS as an antigen delivery platform of heterologous antigens by providing a safer, non-replicating vehicle for vaccination against infections in which this type of response is crucial for protection. In addition, this system may provide an effective strategy to prime DCs ex vivo for immunotherapy against infectious diseases and cancer. Bacterial strains and growth conditions All bacterial strains used in this study are derivatives of Salmonella enterica serovar Typhimurium ( S. Typhimurium) SL1344 and are listed in Supplementary Table S3 . The minD :: cat mutant allele was introduced into S. typhimurium as previously described [39] . All plasmids used in this study were constructed using standard recombinant DNA techniques and are detailed in Supplementary Table S4 . All S. Typhimurium strains were grown in Luria broth containing 0.3 M NaCl to induce the expression of the T3SS encoded on the Salmonella pathogenicity island -1 (SPI-1). Minicell purification Minicells were purified using protocols adapted from previously published methods [23] with several modifications ( Supplementary Fig. S1 ). Briefly, a 500-ml culture of a minD::cat mutant strain was grown under low aeration and agitation until an OD at A 600 of 1.1 was reached. Minicells were subsequently enriched in a series of two low-speed centrifugations at 2,000 g in which the supernatants were collected while the pellets containing mostly bacterial rods were discarded. Minicells were recovered by a final centrifugation for 30 min at 10,000 g , resuspended in a solution of buffered saline gelatin and applied to the top of a continuous 5–20% iodixanol (OptiPrep, Axis-Shield PLC, Scotland) density gradient formed using the gradient forming function of the Gradient Station (Biocomp Instruments; Fredericton, NB, Canada) in SW28 (Beckman Coulter) tubes. Gradients were subjected to 20 min of centrifugation at 2,000 g in a Beckman Coulter ultracentrifuge. After centrifugation, minicell-enriched fractions were collected using the fraction collection feature of the Gradient Station (Biocomp Instruments) in 1.5 ml aliquots. Minicells in the different fractions were pelleted at 18,000 g and resuspended in the appropriate buffer for further usage. Minicells suspended in glycerol were enumerated using DIC microscopy on a CELL-VU disposable slide that contains a chamber of a known depth of 20 μm. The number of contaminating rods in the purified minicell fractions was determined by counting the colony forming units of serial dilutions of the different fractions. The outlined protocol yielded minicells with a diameter of 200 to 550 nm (with an average of 394±90 nm). The average yield of purified minicells was 1.67±0.70 × 10 12 minicells per preparation. The contamination from bacterial rods was estimated to be 1 rod in 10 6 minicells, which represents 0.001% of the total protein mass present in the minicell preparation ( Supplementary Fig. S4 ). This low level of contaminating rods did not impact any of the assays conducted with minicells as proteins potentially secreted by these number of rods would be well below detection in secretion ( Supplementary Fig. S5 ) or antigen presentation ( Supplementary Fig. S6 ) assays. SDS-Polyacrylamide Gel Electrophoresis and Immunoblotting Lysates were solubilized in laemmli buffer and then separated on sodium dodecyl sulphate (SDS)-10 or 15% polyacrylamide gels. The gels were subsequently visualized by Coomassie brilliant blue staining. For immunoblotting, proteins were transferred onto PVDF or nitrocellulose membranes and treated with mouse monoclonal antibodies against the relevant proteins or epitope tags as indicated ( Supplementary Table S5 ). Protein bands were visualized using an Odyssey infrared imaging system (LI-COR Biosciences). When comparing protein concentrations between different samples by immunoblot, all samples were first normalized to the detected integrated intensity of cell lysates after Coomassie blue staining using the Odyssey infrared imaging system ( Supplementary Fig. S3 ). Mass spectrometry analysis Equivalent protein concentrations of minicell and bacterial rod proteins from a parental strain grown under SPI-1 T3SS-inducing conditions were briefly separated on a 10% SDS–PAGE gel and processed for liquid chromatography–tandem mass spectrometry (LC-MS/MS) to identify peptides as previously described [40] . See Supplementary Methods for additional details on data analysis. Electron microscopy Minicells were purified from bacterial rods grown under SPI-1 T3SS-inducing conditions. After purification, the minicells were subsequently osmotically shocked and visualized under the electron microscope following a protocol adapted from Kubori et al. [29] . Immunofluorescence staining Purified minicells were isolated from bacterial rods grown to an optical density measured at 600 nm (OD600) of 1.1. These minicells were serially diluted and spun at 750 g onto acid washed, poly- D lysine coated coverslips and fixed for 30 min in a 4% paraformaldehyde solution in PBS. Coverslips were washed and incubated with a solution of 3% bovine serum albumin in PBS for 30 min. Minicells were subsequently labelled with rabbit polyclonal anti-S. Typhimurium lipopolysaccharide (Difco Laboratories) at a 1:2,000 dilution or mouse monoclonal anti-Flag M2 (Sigma) at a 1:10,000 dilution for 1 h. Minicells were then labelled with secondary anti-rabbit antibody conjugated to Alexa 594, an anti-mouse antibody conjugated to Alexa 488 at a dilution of 1:2,000, and DAPI. Images were captured with a fluorescence microscope (Nikon Diaphot) equipped with a Princeton Instruments CCD camera and analysed using ImageJ (US National Institutes of Health, Bethesda, Maryland, USA). The proportion of minicells expressing SipD on their surface was determined after overlaying captured images showing the LPS stain, the SipD stain and the DIC image of the minicells. For each minicell sample, three different experiments (that is, biological replicates) were used for immunofluorescence analysis and two different fields of view were analysed per biological replicate counting a minimum of 4,000 minicells for each condition. Analysis of T3SS function in bacterial minicells Minicells were purified from a strain carrying plasmids expressing SopB and its chaperone SigE under the control of an arabinose-inducible promoter ( pBAD-sopB-sigE ) and [41] a plasmid expressing HilA. Purified minicells were then incubated for 3 h at 37 °C in the presence of the 0.1% arabinose to allow further expression of the SopB construct. Minicells were subsequently pelleted at 20,000 × g for 30 min at 4 °C, supernatants removed and filtered through a 0.22-μm-pore-size filter to remove any remaining minicells. Proteins from this supernatant were precipitated by adding 0.1% sodium deoxycholate and 10% trichloroacetic acid. After incubation at 4 °C overnight, proteins were recovered by centrifugation at 20,000 g for 20 min. Pellets were washed in acetone, dried and resuspended in Laemmli buffer. Polyacrylamide gel electrophoresis and western blot analysis of the recovered supernatant proteins was carried out as described above. Minicell-mediated protein translocation into cultured cells was assayed as previously described [27] with some modifications. Purified minicells were added to Henle-407 cells grown to ~80% confluency in 15 cm tissue culture dishes in the presence of the proteasome inhibitor MG132 (to prevent effector protein degradation) and 0.2% arabinose. After 2.5 h treatment, the supernatant and extracellular minicells were removed and centrifuged at 8,000 g for 30 min at 4 °C, the supernatant was collected an filtered through a 0.22-μm-pore-size filter to remove any remaining minicells. Henle-407 cells were washed with PBS three times and scraped off the plates in the presence of 5 μM protease inhibitors and 0.1% Triton-X 100. The Triton-X 100 insoluble fraction was resuspended in Laemmli buffer and proteins in the extracellular supernatant and Triton-X 100 soluble fraction were precipitated by addition of ammonium sulphate (50% weight per vol final concentration), resuspended in 10 M Urea, and analysed by western blot analysis. Antigen presentation assay Analysis of antigen delivery and subsequent CD8 + T-cell activation was carried out using an in vitro T-cell activation assay adapted from previously published protocols [2] , [34] with minor modifications detailed in the Supplementary Methods . Adoptive transfer and animal immunization Adoptive transfer experiments were carried out as previously described [42] with minor modification detailed in the Supplementary Methods . For protection studies, BMDCs were prepared from Balb/c mice as outlined in Supplementary Methods , and incubated in the presence of GM-CSF with purified minicells prepared from different bacterial strains, all carrying the Δ asd mutation (to prevent replication of the minor contaminating bacterial rod fraction). The BMDCs were extensively washed and applied in the tail vein of Balb/c recipient mice. Six days after BMDC transfer, mice were challenged i.v. with 7 × 10 3 cfus Listeria monocytogenes strain 10403s and killed 3 days later. Spleens were removed from the killed mice and c.f.u. enumerated by plating dilutions of homogenized tissues. Measurement of OVA-specific CD8 + T-cell responses Splenocytes prepared from immunized mice were resuspended in PBS containing 0.1% BSA and added to a 96-well U-bottom plates at a concentration of 1–2 × 10 6 cells in 50 μl per well. Splenocytes were then stained with conjugated antibodies directed at CD8 (FITC) and CD45.2 (APC), using standard procedures at 4 °C (conjugated antibodies from eBioscience). Stained cells were fixed in 2.5% formaldehyde in PBS at 4 °C overnight and analysed using a FACSCalibur flow cytometer (Becton-Dickson) and FlowJo software (Tree Star, Inc.). All animal experiments were carried out in accordance with and have been approved by the Institutional Animal Care and Use Committee of Yale University. How to cite this article: Carleton, HA. et al. Engineering the type III secretion system in non-replicating bacterial minicells for antigen delivery. Nat. Commun. 4:1590 doi: 10.1038/ncomms2594 (2013).